25-hydroxycholesterol contributes to cerebral inflammation of X-linked adrenoleukodystrophy through activation of the NLRP3 inflammasome X-linked adrenoleukodystrophy (X-ALD), caused by an ABCD1 mutation, is a progressive neurodegenerative disorder associated with the accumulation of very long-chain fatty acids (VLCFA). Cerebral inflammatory demyelination is the major feature of childhood cerebral ALD (CCALD), the most severe form of ALD, but its underlying mechanism remains poorly understood. Here, we identify the aberrant production of cholesterol 25-hydroxylase ( CH25H ) and 25-hydroxycholesterol (25-HC) in the cellular context of CCALD based on the analysis of ALD patient-derived induced pluripotent stem cells and ex vivo fibroblasts. Intriguingly, 25-HC, but not VLCFA, promotes robust NLRP3 inflammasome assembly and activation via potassium efflux-, mitochondrial reactive oxygen species (ROS)- and liver X receptor (LXR)-mediated pathways. Furthermore, stereotaxic injection of 25-HC into the corpus callosum of mouse brains induces microglial recruitment, interleukin-1β production, and oligodendrocyte cell death in an NLRP3 inflammasome-dependent manner. Collectively, our results indicate that 25-HC mediates the neuroinflammation of X-ALD via activation of the NLRP3 inflammasome. X-linked adrenoleukodystrophy (X-ALD) is an inherited metabolic disorder caused by a loss of function mutation in the ATP-binding cassette transporter subfamily D member 1 ( ABCD1 ) gene [1] . ABCD1 mediates the transport of saturated very long-chain fatty acids (VLCFA) from the cytosol to the peroxisome for degradation [2] . Dysfunctional ABCD1, therefore, leads to the accumulation of VLCFA particularly in the adrenal cortex, central nervous system and plasma as well [3] , [4] . While abnormal accumulation of VLCFA is considered an important marker for X-ALD [5] , [6] , how VLCFA is involved in the pathogenesis of X-ALD remains to be clarified. The main manifestation of X-ALD is milder axonopathy of the spinal cord and more severe cerebral inflammatory demyelination [7] . The most severe phenotype of X-ALD is childhood cerebral ALD (CCALD), which is accompanied by acute inflammatory demyelination of the central nervous system that leads to a vegetative state or death within 3–5 years of onset [8] . On the other hand, adrenomyeloneuropathy (AMN), the most prevalent phenotype, manifests as a slowly progressive myelopathy in the adulthood [7] , [9] . The presence of cerebral inflammation is a significant symptom of CCALD, but how cerebral inflammation is initiated or promoted in CCALD patients is still poorly understood. Nevertheless, abnormal accumulation of VLCFA is considered as a biochemical trigger for the pathophysiology of CCALD including cerebral inflammatory response [10] . Furthermore, the pathogenesis of cerebral ALD could be affected by a range of genetic and environmental factors [9] . Although Abcd1 -deficient mice exhibited an increased level of VLCFA in the brain and adrenal gland, these mice did not show any characteristics of CCALD phenotypes including the cerebral pathology [11] . Thus, this lack of CCALD phenotype in Abcd1 -deficient mice makes it more difficult to study the molecular basis of cerebral inflammation of CCALD caused by VLCFA accumulation. A dysregulated innate immune response has been increasingly considered a potential contributor to cerebral inflammation and neurodegenerative disorders [12] . Of particular interest, nucleotide-binding oligomerization domain-like (NOD-like) receptor containing pyrin domain 3 (NLRP3) inflammasome signalling has been proposed as a crucial mediator in the progression of Alzheimer’s diseases [13] , [14] . The inflammasome is a caspase-1-activating multi-protein complex that, once assembled, leads to the production of key pro-inflammatory cytokines interleukin-1β (IL-1β) and IL-18 (ref. 15 ). Unlike the other identified inflammasomes, NLRP3 can be activated by a wide range of stimulators from microbial toxin to host endogenous metabolites such as palmitate, cholesterol crystals and amyloid β (refs 15 , 16 ). On the basis of its potent recognition capability under diverse stress conditions, NLRP3 is thought to be a crucial sensor of cellular abnormalities to initiate inflammation. The robust expression of the NLRP3 inflammasome components in mouse brain microglia was reported previously [17] . Of particular interest, Nlrp3 -deficient mice exhibited delayed demyelination and oligodendrocyte depletion in a cuprizone-induced demyelination model [18] . In the present study, we used microarray analysis and identified 25-hydroxycholesterol (25-HC) as a potent mediator in the pathogenesis of X-ALD. Our data suggest that 25-HC, but not VLCFA, contributes to the cerebral inflammation of X-ALD via activation of the NLRP3 inflammasome pathway. CH25H upregulation in CCALD patient-derived cells To recapitulate the distinctive features of X-ALD phenotypes, we have previously generated induced pluripotent stem cells (iPSCs) from the fibroblasts of healthy control and X-ALD patients including those with CCALD and AMN [19] . In early passage cultures of iPSCs, VLCFA levels were significantly higher in CCALD-iPSCs compared with control iPSCs, AMN-iPSCs or human embryonic stem cells (hESCs) ( Supplementary Fig. 1 ). To gain molecular insight into the inflammatory phenotype of CCALD, we performed microarray-based transcriptional profiling analysis of hESCs, control-, AMN- and CCALD-iPSCs. We then identified 40 up- and 30 downregulated genes in the CCALD-iPSCs compared with control iPSCs ( Supplementary Fig. 2 ). Among the 40 significantly upregulated genes, the expression level of nine genes was positively correlated with phenotypic severity in the following order (control<AMN<CCALD) ( Fig. 1a ). We also selected five candidate genes from 40 up- and 30 downregulated genes based on functional categorization of lipid metabolic processes for their potential implication in VLCFA accumulation. Venn diagram analysis indicated that CH25H (cholesterol 25-hydroxylase) and CAT (catalase) were simultaneously relevant to the phenotypic severity and lipid metabolism categories ( Fig. 1b ). CH25H is a hydroxylating enzyme that converts cholesterol to 25-hydroxycholesterol (25-HC) [20] , whereas CAT is a well-known antioxidant enzyme that catalyses the decomposition of hydrogen peroxide [21] . Given that oxysterols such as 25-HC are involved in the regulation of inflammation and also positively implicated in the pathogenesis of inflammatory or neurodegenerative diseases [22] , [23] , [24] , CH25H was then selected and examined for its potential role in the cerebral inflammatory phenotype of X-ALD. 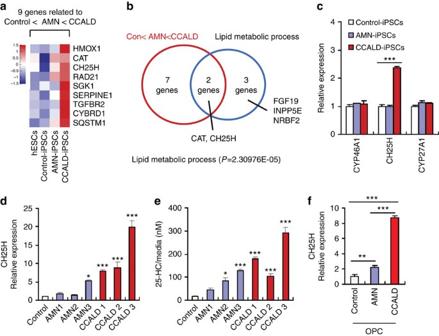Figure 1:CH25His upregulated in CCALD patient-derived cells. (a) Candidate genes significantly up- or downregulated (fold-change cutoff ≥2 andP<0.05) were selected based on the microarray analysis of human ESCs, control-, AMN- and CCALD-iPSCs. Heat map of nine selected genes showing the expression patterns correlated with disease severity via microarray analysis. (b) Venn diagram of overlapping genes between nine genes related to disease severity and five genes (among 70 genes) related to lipid metabolism. Catalase (CAT) andCH25Hbelong to both categories. (c) Relative mRNA expression of three cholesterol-hydroxylating enzymes in the control- and AMN- or CCALD-iPSCs measured by quantitative real-time PCR analysis. (n=6) (d,e) Levels ofCH25HmRNA in the cell lysates (d) and of 25-HC in the culture supernatants (e) of control- (human dermal fibroblast), 3 AMN- and 3 CCALD-fibroblasts. (d,n=6;e,n=4) (f) Relative mRNA expression ofCH25Hin the control- or X-ALD-iPSC-derived oligodendrocyte precursor cells (AMN- or CCALD-OPCs). (n=6) For all panels, *P<0.05, **P<0.01 and ***P<0.001. Figure 1: CH25H is upregulated in CCALD patient-derived cells. ( a ) Candidate genes significantly up- or downregulated (fold-change cutoff ≥2 and P <0.05) were selected based on the microarray analysis of human ESCs, control-, AMN- and CCALD-iPSCs. Heat map of nine selected genes showing the expression patterns correlated with disease severity via microarray analysis. ( b ) Venn diagram of overlapping genes between nine genes related to disease severity and five genes (among 70 genes) related to lipid metabolism. Catalase ( CAT ) and CH25H belong to both categories. ( c ) Relative mRNA expression of three cholesterol-hydroxylating enzymes in the control- and AMN- or CCALD-iPSCs measured by quantitative real-time PCR analysis. ( n =6) ( d , e ) Levels of CH25H mRNA in the cell lysates ( d ) and of 25-HC in the culture supernatants ( e ) of control- (human dermal fibroblast), 3 AMN- and 3 CCALD-fibroblasts. ( d , n =6; e , n =4) ( f ) Relative mRNA expression of CH25H in the control- or X-ALD-iPSC-derived oligodendrocyte precursor cells (AMN- or CCALD-OPCs). ( n =6) For all panels, * P <0.05, ** P <0.01 and *** P <0.001. Full size image In addition to CH25H, CYP46A1 (also known as cholesterol 24-hydroxylase) and CYP27A1 are other major oxysterol-producing enzymes that produce 24-HC and 27-HC, respectively [22] . However, the expression of CYP46A1 or CYP27A1 was not significantly altered in CCALD-iPSCs according to microarray analysis ( Supplementary Table 1 ). Increased mRNA expression of CH25H was also validated in the CCALD-iPSCs by quantitative real-time PCR analysis, while the expression of CYP46A1 and CYP27A1 was similar in all three cell types ( Fig. 1c ). To further validate the increased expression of CH25H of CCALD patients-derived cells, we compared the levels of CH25H in the ex vivo primary fibroblasts of healthy control, AMN patients and CCALD patients. Consistent with the expression pattern of iPSCs, all three CCALD patients’ fibroblasts showed a significant increase in CH25H mRNA expression compared with control fibroblasts ( Fig. 1d ). In addition, significant upregulation of CH25H mRNA was observed in one AMN fibroblast, but not in two other AMN fibroblasts ( Fig. 1d ). Similarly, the level of 25-HC, a product of CH25H, also was significantly increased in the culture supernatants of all CCALD fibroblast cultures compared with control fibroblast cultures ( Fig. 1e ). To confirm the potential relevance of this finding in oligodendrocytes, which is the cell type primarily affected in the demyelination process of X-ALD, we generated oligodendrocyte precursor cells (CCALD-OPCs) differentiated from CCALD-iPSCs ( Supplementary Fig. 3 ). Consistent with the above observations, CH25H mRNA levels were significantly higher in CCALD-OPCs than control- or AMN-OPCs ( Fig. 1f ). These findings strongly demonstrate that the expression of CH25H is significantly upregulated in CCALD-derived cells. ABCD1-dependent regulation of CH25H mRNA expression To determine whether a defect in function of ABCD1 was involved in the induction of CH25H mRNA expression, we reduced ABCD1 expression in control fibroblasts by siRNA-mediated knockdown ( Supplementary Fig. 4a ). Knockdown of ABCD1 caused a significant increase in VLCFA levels and CH25H mRNA expression ( Fig. 2a,b ). Of note, CCALD-fibroblasts showed much higher levels of VLCFA and of CH25H mRNA than ABCD1-knockdowned fibroblasts ( Fig. 2a,b ). Conversely, ectopic expression of ABCD1 in CCALD-fibroblasts significantly attenuated the level of VLCFA and CH25H mRNA ( Supplementary Fig. 4b and Fig. 2c,d ). These findings indicate that the dysfunction of ABCD1 observed in X-ALD patients contributes to the induction of CH25H expression. Supporting these observations, increased Ch25h expression was also found in the brain homogenates of Abcd1 -deficient mice compared with wild-type mice, while the expression of other cholesterol-metabolizing enzymes was unchanged ( Fig. 2e ). 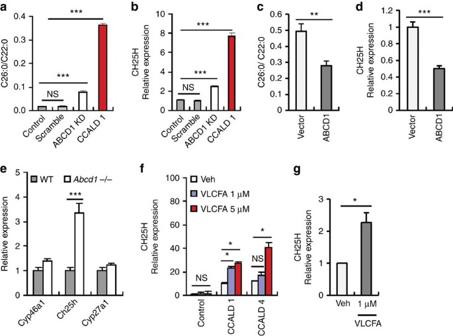Figure 2: ABCD1 regulates the induction ofCH25Hexpression in a VLCFA-dependent manner. (a,b) Cellular levels of VLCFA (a) and mRNA levels ofCH25H(b) in control fibroblasts untransfected or transfected with scrambled- orABCD1-targeting siRNA (ABCD1 KD) and in CCALD1 fibroblasts. (n=6) (c,d) Cellular levels of VLCFA (c) and mRNA levels ofCH25H(d) in CCALD1 fibroblasts infected with lentiviral particles expressing empty vector orABCD1gene. (n=5) (e) Relative mRNA expression ofCyp46a1,Ch25handCyp27a1in the brain homogenates of WT orAbcd1-deficient mice. (n=6). (f,g) Relative mRNA levels ofCH25Hin control- or two CCALD-fibroblasts (f) and in CCALD-OPCs (g) treated with vehicle (0.05% DMSO in PBS) or VLCFA at indicated concentration for 3 h. (f,n=6;g,n=5) For all panels, *P<0.05, **P<0.01, and ***P<0.001. NS, not significant. Figure 2: ABCD1 regulates the induction of CH25H expression in a VLCFA-dependent manner. ( a , b ) Cellular levels of VLCFA ( a ) and mRNA levels of CH25H ( b ) in control fibroblasts untransfected or transfected with scrambled- or ABCD1 -targeting siRNA (ABCD1 KD) and in CCALD1 fibroblasts. ( n =6) ( c , d ) Cellular levels of VLCFA ( c ) and mRNA levels of CH25H ( d ) in CCALD1 fibroblasts infected with lentiviral particles expressing empty vector or ABCD1 gene. ( n =5) ( e ) Relative mRNA expression of Cyp46a1 , Ch25h and Cyp27a1 in the brain homogenates of WT or Abcd1 -deficient mice. ( n =6). ( f , g ) Relative mRNA levels of CH25H in control- or two CCALD-fibroblasts ( f ) and in CCALD-OPCs ( g ) treated with vehicle (0.05% DMSO in PBS) or VLCFA at indicated concentration for 3 h. ( f , n =6; g , n =5) For all panels, * P <0.05, ** P <0.01, and *** P <0.001. NS, not significant. Full size image Next, we examined whether VLCFA accumulation triggered by ABCD1 dysfunction directly mediated the induction of CH25H expression. Exogenous addition of VLCFA did not affect the expression of CH25H in control fibroblasts, possibly due to the presence of a fully functional ABCD1 , but led to significantly increased CH25H mRNA levels in CCALD-fibroblasts ( Fig. 2f ). Similarly, VLCFA treatment also led to increased expression of CH25H in CCALD-OPCs ( Fig. 2g ). These observations demonstrate that the accumulation of VLCFAs resulting from a defective ABCD1 gene may account for the induction of CH25H expression in CCALD-derived cells. Microglial recruitment and IL-1β production by 25-HC Recently, much attention has been paid to oxysterols, including 25-HC, as a potential regulator of innate or adaptive immune responses [23] , [24] , [25] . Given that neuroinflammation is closely related to the pathogenesis of CCALD [7] , we examined whether the elevated level of 25-HC could mediate cerebral inflammation. Therefore, we stereotactically injected 25-HC into the corpus callosum of wild-type mouse brains ( Fig. 3a ), and measured the recruitment of microglia, a major cell type for inducing neuroinflammation. To our surprise, significant recruitment of Iba-1-positive microglia was observed around the 25-HC-injected region, but not around the contralateral vehicle-injected region ( Fig. 3b,c ). Then, we examined whether 25-HC could mediate pro-inflammatory responses. Considering that pro-inflammatory cytokines such as TNF-α, IL-1β and IFN-γ were increased in the demyelination plaques of X-ALD brains [3] , [26] , these pro-inflammatory cytokines were measured in mouse brain homogenates. Among the tested cytokines, only IL-1β production was significantly increased in the 25-HC-injected hemisphere compared with the contralateral control region ( Fig. 3d ), whereas the levels of other pro-inflammatory cytokines such as TNF-α, IFN-γ, IL-6 and MCP-1 were unchanged in the two regions ( Supplementary Fig. 5 ). 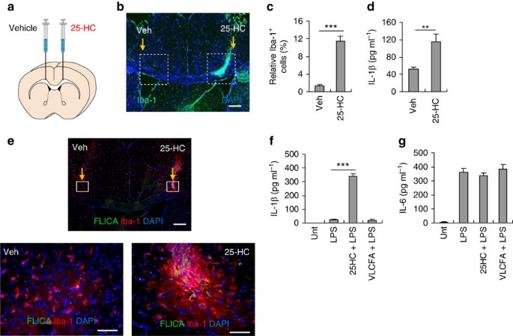Figure 3: 25-HC induces microglial recruitment and IL-1β production. (a) Illustration of stereotaxic injection of 25-HC (100 μM) or vehicle (0.1% ethanol in PBS) into the corpus callosum of mouse brain. (b) Representative immunofluorescence image of a coronal brain section stained with anti-Iba-1 antibody (green). DAPI represents the nuclear signal (blue). Scale bar, 200 μm. (c) Quantification of Iba-1-positive cells in the boxed areas of vehicle- or 25-HC-injected regions inb. (n=8) (d) Quantification of IL-1β in the brain homogenates of vehicle- or 25-HC-injected hemisphere. (n=11) (e) Representative immunofluorescence image of brain section co-stained with FLICA (green) and anti-Iba-1 antibody (red) after injection of vehicle or 25-HC. Magnified immunofluorescence images of the boxed areas in the upper panel are displayed in the lower panel: 25-HC-injected area (right) or vehicle-injected area (left). Scale bars, 200 μm (upper); or 50 μm (lower). (f,g) Quantification of IL-1β or IL-6 in the culture supernatants of mouse BMDMs untreated or treated with 25-HC (70 μM) or VLCFA (70 μM) for 10 h in the presence of LPS (0.25 μg ml−1, last 4 h) as indicated. (n=6). For all panels, **P<0.01 and ***P<0.001. Figure 3: 25-HC induces microglial recruitment and IL-1β production. ( a ) Illustration of stereotaxic injection of 25-HC (100 μM) or vehicle (0.1% ethanol in PBS) into the corpus callosum of mouse brain. ( b ) Representative immunofluorescence image of a coronal brain section stained with anti-Iba-1 antibody (green). DAPI represents the nuclear signal (blue). Scale bar, 200 μm. ( c ) Quantification of Iba-1-positive cells in the boxed areas of vehicle- or 25-HC-injected regions in b . ( n =8) ( d ) Quantification of IL-1β in the brain homogenates of vehicle- or 25-HC-injected hemisphere. ( n =11) ( e ) Representative immunofluorescence image of brain section co-stained with FLICA (green) and anti-Iba-1 antibody (red) after injection of vehicle or 25-HC. Magnified immunofluorescence images of the boxed areas in the upper panel are displayed in the lower panel: 25-HC-injected area (right) or vehicle-injected area (left). Scale bars, 200 μm (upper); or 50 μm (lower). ( f , g ) Quantification of IL-1β or IL-6 in the culture supernatants of mouse BMDMs untreated or treated with 25-HC (70 μM) or VLCFA (70 μM) for 10 h in the presence of LPS (0.25 μg ml −1 , last 4 h) as indicated. ( n =6). For all panels, ** P <0.01 and *** P <0.001. Full size image IL-1β is a key inflammatory cytokine that triggers pro-inflammatory responses at the site of inflamed tissues [27] . Unlike other cytokines, the production of functional IL-1β requires the additional post-translational regulator, caspase-1 (ref. 28 ). Thus, to validate whether the elevated level of IL-1β in the 25-HC-injected region resulted from the potentiated activation of caspase-1, we examined the presence of active caspase-1 in the corpus callosum of mouse brain using an active caspase-1-specific fluorochrome-labeled inhibitors of caspases (FLICA) probe, which yields green fluorescence in active-caspase-1-containing cells. Active caspase-1 was evident only in the microglia in the 25-HC-injected region ( Fig. 3e ), which indicated that the elevated IL-1β reflected the robust activation of caspase-1. Furthermore, an amoeboid morphology of the activated microglia was observed around the 25-HC-injected regions ( Fig. 3e , lower right). To further confirm whether 25-HC could trigger the production of IL-1β in cell culture, we examined the potential effect of 25-HC and VLCFA in mouse bone marrow-derived macrophages (BMDMs). Intriguingly, 25-HC, but not VLCFA, in the presence of lipopolysaccharide (LPS) co-treatment caused a marked secretion of IL-1β in BMDMs ( Fig. 3f ), whereas neither 25-HC nor VLCFA affected the LPS-stimulated secretion of IL-6 ( Fig. 3g ). However, 25-HC treatment did not induce mRNA expression of lL-1β and IL-6 in BMDMs ( Supplementary Fig. 6a,b ). These observations suggest that 25-HC, but not VLCFA, could activate the production of IL-1β in a transcription-independent manner. NLRP3 inflammasome assembly and activation by 25-HC Activation of caspase-1 requires the assembly and activation of the inflammasome complex [15] . This led us to investigate whether heightened 25-HC production could activate inflammasome signalling. Consistent with the above results, 25-HC treatment promoted a robust processing of caspase-1 and secretion of active IL-1β in mouse BMDMs and microglia in the presence of LPS co-treatment ( Fig. 4a ). This 25-HC-triggered activation of caspase-1 and IL-1β was also found in mouse primary mixed glial cells and human THP-1 macrophages ( Supplementary Fig. 7a,b ). In contrast, VLCFA did not activate caspase-1 signalling in BMDMs ( Fig. 4b ), mixed glial cells, or THP-1 cells ( Supplementary Fig. 8a,b ), which demonstrated that caspase-1-activating capability was specific to 25-HC, but not to VLCFA. In particular, the microglia-enriched population exhibited a stronger activation of caspase-1 signalling than mixed glial cells containing <10% microglia ( Supplementary Fig. 9a,b ). Indeed, the expression of the major inflammasome components, apoptosis-associated speck-like protein containing a caspase-recruitment domain (ASC) and NLRP3, were increased in the microglia relative to mixed glial cells ( Supplementary Fig. 9b ). These data suggest that microglia might be the primary cell population that activates caspase-1 when 25-HC accumulates in the brain. 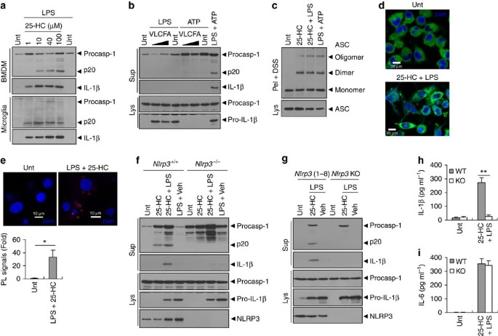Figure 4: 25-HC promotes the assembly and activation of the NLRP3 inflammasome. (a) Immunoblots of culture supernatants from mouse BMDMs and microglia untreated or treated with 25-HC (10 h) in the presence of LPS (last 4 h). (b) Immunoblots from BMDMs untreated or treated with VLCFA (40 or 100 μM, 10 h) in the presence of LPS (last 4 h) or ATP (2.5 mM, last 45 min), or primed with LPS (3 h), followed by ATP. (c) Immunoblots of DSS-crosslinked pellets (pel + DSS) or cellular lysates (Lys) from BMDMs untreated or treated with 25-HC in the presence of LPS, or treated with LPS, followed by ATP. (d) Confocal images of NLRP3-GFP-expressing macrophages untreated or treated with 25-HC (50 μM, 10 h) in the presence of LPS. DAPI represents the nuclear signal (blue). Scale bars, 10 μm. (e) Proximity-ligation (PL) assay of NLRP3 and ASC in BMDMs treated with 25-HC (50 μM, 10 h) in the presence of LPS. PL signals (red) represent the molecular association of NLRP3 and ASC. Data are shown as a representative image from five-independent samples (upper panel). DAPI represents the nuclear signal (blue). Scale bars, 10 μm. Relative intensity of PL signals (per DAPI signals) was determined and is displayed in the lower panel. (n=5) (f)Nlrp3+/+orNlrp3−/−BMDMs were treated with 25-HC (100 μM) or vehicle (0.1% ethanol in PBS) in the presence of LPS (last 4 h) as indicated, and analysed by immunoblot. (g)Nlrp3-expressing (1–8) orNlrp3-deficient immortalized BMDMs were treated with 25-HC in the presence of LPS as indicated and analysed by immunoblot. (h,i) Quantification of IL-1β (h) or IL-6 (i) in supernatant fractions ofNlrp3+/+(WT) orNlrp3−/−(KO) microglial cells treated with 25-HC (50 μM) in the presence of LPS. (n=5) (b,c,f,g) Culture supernatants (Sup), cellular lysates (Lys) or DSS-crosslinked pellets (Pel + DSS) as indicated were analysed by immunoblot. For all panels, *P<0.05 and **P<0.01. Figure 4: 25-HC promotes the assembly and activation of the NLRP3 inflammasome. ( a ) Immunoblots of culture supernatants from mouse BMDMs and microglia untreated or treated with 25-HC (10 h) in the presence of LPS (last 4 h). ( b ) Immunoblots from BMDMs untreated or treated with VLCFA (40 or 100 μM, 10 h) in the presence of LPS (last 4 h) or ATP (2.5 mM, last 45 min), or primed with LPS (3 h), followed by ATP. ( c ) Immunoblots of DSS-crosslinked pellets (pel + DSS) or cellular lysates (Lys) from BMDMs untreated or treated with 25-HC in the presence of LPS, or treated with LPS, followed by ATP. ( d ) Confocal images of NLRP3-GFP-expressing macrophages untreated or treated with 25-HC (50 μM, 10 h) in the presence of LPS. DAPI represents the nuclear signal (blue). Scale bars, 10 μm. ( e ) Proximity-ligation (PL) assay of NLRP3 and ASC in BMDMs treated with 25-HC (50 μM, 10 h) in the presence of LPS. PL signals (red) represent the molecular association of NLRP3 and ASC. Data are shown as a representative image from five-independent samples (upper panel). DAPI represents the nuclear signal (blue). Scale bars, 10 μm. Relative intensity of PL signals (per DAPI signals) was determined and is displayed in the lower panel. ( n =5) ( f ) Nlrp3 +/+ or Nlrp3 −/− BMDMs were treated with 25-HC (100 μM) or vehicle (0.1% ethanol in PBS) in the presence of LPS (last 4 h) as indicated, and analysed by immunoblot. ( g ) Nlrp3 -expressing (1–8) or Nlrp3 -deficient immortalized BMDMs were treated with 25-HC in the presence of LPS as indicated and analysed by immunoblot. ( h , i ) Quantification of IL-1β ( h ) or IL-6 ( i ) in supernatant fractions of Nlrp3 +/+ (WT) or Nlrp3 −/− (KO) microglial cells treated with 25-HC (50 μM) in the presence of LPS. ( n =5) ( b , c , f , g ) Culture supernatants (Sup), cellular lysates (Lys) or DSS-crosslinked pellets (Pel + DSS) as indicated were analysed by immunoblot. For all panels, * P <0.05 and ** P <0.01. Full size image To provide molecular insight into the inflammasome activation by 25-HC, we next investigated ASC oligomerization, which is a critical step in inflammasome activation [29] . Consistent with the above data showing the secretion of active caspase-1 and IL-1β, 25-HC promoted a robust oligomerization of ASC as determined by a discuccinimidyl suberate (DSS)-crosslinking assay ( Fig. 4c ). Among the identified inflammasomes, NLRP3 shows the unique features of recognizing diverse endogenous danger signals such as palmitic acid [16] , [30] . To investigate the possibility that 25-HC could activate the NLRP3 inflammasome, we examined the oligomerization of NLRP3 using NLRP3-GFP-expressing macrophages. Noticeably, 25-HC treatment caused formation of speck-like aggregates of NLRP3 ( Fig. 4d ), indicating that 25-HC might act as another endogenous danger signal for NLRP3 activation. To further validate whether 25-HC could trigger the assembly of NLRP3 inflammasome, the spatial proximity of NLRP3 with ASC was measured using a proximity-ligation assay as recently described [31] . Consistent with the oligomerization of ASC and NLRP3, 25-HC treatment caused a marked increase in the proximity-ligation signal, which represented the molecular assembly of NLRP3 with ASC ( Fig. 4e and Supplementary Fig. 10 ). Supporting these observations, 25-HC-promoted caspase-1 processing and IL-1β secretion were completely abolished in Nlrp3 -deficient BMDMs ( Fig. 4f ), microglia and mixed glial cells ( Supplementary Fig. 11a,b ). Conversely, the restoration of NLRP3 expression in Nlrp3 −/− immortalized BMDMs regained the susceptibility to 25-HC-induced caspase-1 activation ( Fig. 4g ). In correlation with these findings, 25-HC-triggered IL-1β secretion was largely impaired in Nlrp3 -lacking microglia ( Fig. 4h ) and BMDMs ( Supplementary Fig. 11c ), while LPS-triggered IL-6 secretion was not affected by the absence of NLRP3 in either cell type ( Fig. 4i and Supplementary Fig. 11d ). These data strongly demonstrate that 25-HC is a potent inducer of the NLRP3 inflammasome assembly and activation. Molecular mechanism of NLRP3 activation by 25-HC Despite the fact that diverse stimulators have been shown to activate NLRP3 inflammasomes, the detailed molecular mechanism of how NLRP3 is activated is not fully understood. To provide molecular insight into the NLRP3 activation by 25-HC, we first examined its dependence on potassium (K + ) efflux, currently regarded as the most common mediator of NLRP3 activation in response to diverse stimulators [32] . The inhibition of K + efflux by glibenclamide or high extracellular KCl markedly attenuated 25-HC-induced caspase-1 and IL-1β processing in mouse BMDMs ( Fig. 5a ). Consistently, glibenclamide also blocked the oligomerization of ASC ( Fig. 5b ) and the association of NLRP3 and ASC ( Fig. 5c and Supplementary Fig. 12 ) in mouse BMDMs in response to 25-HC treatment. These findings indicate that K + efflux is involved in the 25-HC-triggered activation of NLRP3 inflammasome. 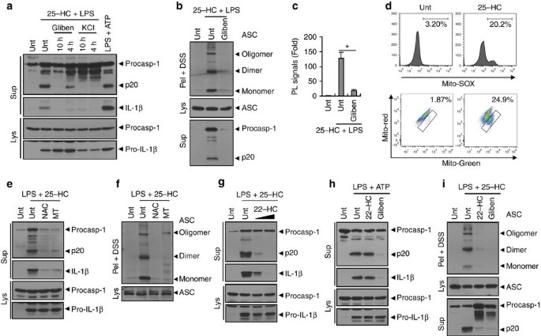Figure 5: 25-HC activates the NLRP3 inflammasome signalling in a potassium efflux/mitochondrial ROS/LXR-dependent manner. (a) Immunoblots of mouse BMDMs treated with 25-HC (50 μM, 10 h) and LPS (final 4 h) in the presence of glibenclamide (50 μM) or KCl (20 mM) for the indicated times, or treated with LPS, followed by ATP. (b) Immunoblots of BMDMs treated with 25-HC (50 μM, 10 h) and LPS (final 4 h) in the presence of glibenclamide (50 μM, 10 h). (c) PL assay of NLRP3 and ASC in microglia similarly treated as inb. Relative PL signals (per DAPI) are displayed. (n=5) *P<0.05 (d) Flow cytometric analysis of BMDMs treated with 25-HC (50 μM, 10 h) and LPS (final 3 h) after staining with MitoSOX (upper panel) or co-stained with MitoTracker Green and MitoTracker Deep Red (lower panel). (e,f) Immunoblots of BMDMs primed with LPS (3 h), followed by treatments with 25-HC (80 μM) in the presence of NAC (20 mM) or Mito-TEMPO (MT, 200 μM) for 6 h. (g,h) Immunoblots of BMDMs primed with LPS (3 h), followed by 25-HC (80 μM) in the presence of 22-HC (50 or 100 μM) for 6 h (g), or primed with LPS in the presence of 22-HC (100 μM) or glibenclamide (50 μM) for 3 h, followed by ATP (2 mM, 45 min) (h). (i) Immunoblots of BMDMs primed with LPS (3 h), followed by 25-HC (80 μM) in the presence of 22-HC (100 μM) or glibenclamide (50 μM) for 6 h. (a,b,e–i) Culture supernatants (Sup), cellular lysates (Lys) or DSS-crosslinked pellets (Pel + DSS) as indicated were analysed by immunoblot. Figure 5: 25-HC activates the NLRP3 inflammasome signalling in a potassium efflux/mitochondrial ROS/LXR-dependent manner. ( a ) Immunoblots of mouse BMDMs treated with 25-HC (50 μM, 10 h) and LPS (final 4 h) in the presence of glibenclamide (50 μM) or KCl (20 mM) for the indicated times, or treated with LPS, followed by ATP. ( b ) Immunoblots of BMDMs treated with 25-HC (50 μM, 10 h) and LPS (final 4 h) in the presence of glibenclamide (50 μM, 10 h). ( c ) PL assay of NLRP3 and ASC in microglia similarly treated as in b . Relative PL signals (per DAPI) are displayed. ( n =5) * P <0.05 ( d ) Flow cytometric analysis of BMDMs treated with 25-HC (50 μM, 10 h) and LPS (final 3 h) after staining with MitoSOX (upper panel) or co-stained with MitoTracker Green and MitoTracker Deep Red (lower panel). ( e , f ) Immunoblots of BMDMs primed with LPS (3 h), followed by treatments with 25-HC (80 μM) in the presence of NAC (20 mM) or Mito-TEMPO (MT, 200 μM) for 6 h. ( g , h ) Immunoblots of BMDMs primed with LPS (3 h), followed by 25-HC (80 μM) in the presence of 22-HC (50 or 100 μM) for 6 h ( g ), or primed with LPS in the presence of 22-HC (100 μM) or glibenclamide (50 μM) for 3 h, followed by ATP (2 mM, 45 min) ( h ). ( i ) Immunoblots of BMDMs primed with LPS (3 h), followed by 25-HC (80 μM) in the presence of 22-HC (100 μM) or glibenclamide (50 μM) for 6 h. ( a , b , e – i ) Culture supernatants (Sup), cellular lysates (Lys) or DSS-crosslinked pellets (Pel + DSS) as indicated were analysed by immunoblot. Full size image In addition to K + efflux, mitochondrial damage or mitochondrial ROS (mtROS) production is also considered a crucial mediator of NLRP3 activation in response to diverse NLRP3 agonists [16] , [33] . Interestingly, 25-HC treatment induced a considerable increase in mtROS-producing cells as measured using a mtROS-specific MitoSOX probe in BMDMs ( Fig. 5d , upper panel). To provide more evidence that 25-HC could impair the function of mitochondria, we determined another indication of mitochondrial damage by co-staining with MitoTracker Green and MitoTracker Deep Red to measure the dissipation of mitochondrial membrane potential [33] , [34] , [35] . Consistent with mtROS production, treatment with 25-HC caused an obvious increase in the damaged mitochondria-containing cell population ( Fig. 5d , lower panel). This increase in mtROS-producing or damaged mitochondria-containing cells was also observed in the Nlrp3 -deficient BMDMs upon 25-HC stimulation ( Supplementary Fig. 13a,b ), indicating that these mitochondrial alterations by 25-HC were not consequences of caspase-1/inflammasome activation. Similarly, 25-HC treatment resulted in the production of mtROS in microglia ( Supplementary Fig. 13a , lower panel). These observations indicate that 25-HC treatment could impair mitochondria in an inflammasome activity-independent manner. Additionally, N -acetyl-cysteine (NAC), a general antioxidant, and Mito-TEMPO, a mitochondria-specific ROS scavenger, led to a marked reduction in caspase-1 activation ( Fig. 5e ) and ASC oligomerization ( Fig. 5f ) in BMDMs stimulated with 25-HC. As expected, Mito-TEMPO considerably attenuated the increase in mtROS-producing BMDMs ( Supplementary Fig. 14a ), suggesting that mtROS production might be related to the underlying mechanism of NLRP3 inflammasome actiation by 25-HC. Of note, the 25-HC-induced mitochondrial alterations were not an immediate, but rather a delayed phenomenon that was observed after at least 3 h of 25-HC treatment ( Supplementary Fig. 14b ). In correlation with this finding, 25-HC-induced caspase-1 activation was observed only after at least 6 h of 25-HC treatment ( Supplementary Fig. 15a,b ). On the basis of these data, we inferred that 25-HC caused the mitochondrial damage in the delayed response, which was likely associated with the NLRP3 activation by 25-HC. A recent report showed that liver X receptor (LXR) ligands, such as TO901317 or 25-HC, promoted the caspase-1-dependent cell death of colon cancer cells [36] . Furthermore, the authors proposed that LXR ligands could induce the activation of NLRP3 inflammasome possibly through inducing the extracellular secretion of ATP [36] . Therefore, we examined the involvement of LXR signalling in the 25-HC-triggered activation of NLRP3 using a LXR antagonist, 22(S)-hydroxycholesterol (22(S)-HC). Co-treatment with 22(S)-HC showed a remarkable reduction of caspase-1 and IL-1β secretion in mouse BMDMs stimulated with 25-HC ( Fig. 5g ). However, 22(S)-HC did not abolish the ATP-stimulated canonical NLRP3 inflammasome activation ( Fig. 5h ). Consistently, 22(S)-HC also blocked the 25-HC-induced oligomerization of ASC ( Fig. 5i ). These data suggest that LXR signalling might be mediated in the 25-HC-triggered activation of NLRP3. In agreement with a recent report [36] , TO901317, another synthetic LXR agonist, exhibited the potent capability to activate caspase-1 ( Supplementary Fig. 16a ). Unlike 25-HC, TO901317-induced caspase-1 activation was observed in Nlrp3 −/− BMDMs ( Supplementary Fig. 16a ) and was not inhibited by the potassium efflux blocker glibenclamide ( Supplementary Fig. 16b ). These observations demonstrate that TO901317 could promote caspase-1 activation in an NLRP3-independent manner. Furthermore, TO901317 exhibited much higher toxicity to BMDMs compared with 25-HC ( Supplementary Fig. 16c ). On the basis of these findings, LXR signalling was potentially involved in NLRP3 inflammasome activation at least in the case of 25-HC stimulation. Supporting our data, the 25-HC-induced secretion of IL-1β was effectively suppressed by the K + efflux blocker, the mtROS scavenger and the LXR antagonist ( Supplementary Fig. 17 ). NLRP3 deficiency reduces cerebral inflammation by 25-HC To validate the contribution of the NLRP3 inflammasome to 25-HC-induced cerebral inflammation, we measured the recruitment of microglia after the stereotaxic injection of 25-HC into the corpus callosum of Nlrp3 +/+ and Nlrp3 −/− mice. Recruitment of microglia into the 25-HC-injected region was significantly reduced in Nlrp3 -deficient mice ( Fig. 6a,b ). Moreover, 25-HC-induced production of IL-1β was significantly attenuated in the brain of Nlrp3 −/− mice ( Fig. 6c ). To further support these data, we used a recombinant IL-1 receptor antagonist (IL-1Ra) to confirm whether microglial recruitment was inflammasome-dependent in our experiments. 25-HC-triggered recruitment of microglia was significantly reduced by the administration of the IL-1Ra ( Fig. 6d,e ), which indicated that IL-1β played a crucial role in the recruitment of microglia into the 25-HC-injected area. 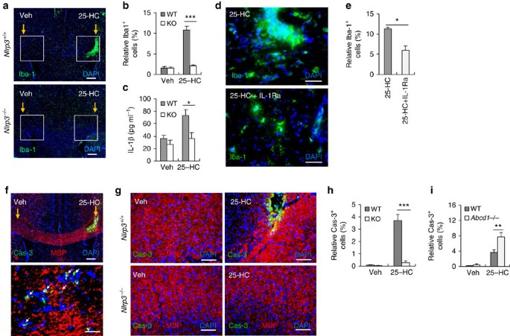Figure 6: 25-HC promotes the microglial recruitment and oligodendrocyte cell death in an NLRP3 inflammasome-dependent manner. (a) Immunohistochemical staining of coronal brain sections with anti-Iba-1 antibody (green) and DAPI (blue) after bilateral stereotaxic injection of 25-HC (100 μM) or vehicle into the brain ofNlrp3+/+orNlrp3−/−mice. Scale bar, 200 μm. (b) Quantification of Iba-1+microglia in confocal images of vehicle- or 25-HC-injected brains fromNlrp3+/+(WT) orNlrp3−/−(KO) mice. (n=6). (c) Quantification of IL-1β in the brain homogenates of vehicle- or 25-HC-injected hemispheres fromNlrp3+/+(WT) orNlrp3−/−(KO) mice. (n=7) (d) Immunohistochemical staining of brain sections with anti-Iba-1 antibody (green) after stereotaxic injection of 25-HC (100 μM) together with recombinant IL-1 receptor antagonist (IL-1Ra, 5 μg). Scale bar, 50 μm. (e) Quantification of Iba-1+microglia in the confocal images of vehicle- or 25-HC-injected brain sections as treated ind. (n=4) (f) Immunohistochemical staining of brain sections with anti-active caspase-3 antibody (green), anti-myelin basic protein antibody (MBP, red), and DAPI (blue). Lower panel is representative magnified image of a 25-HC-injected region. Arrows indicate the active caspase-3-positive oligodendrocytes (yellow). Scale bars, 200 μm (upper); 50 μm (lower). (g) Immunohistochemical staining of brain sections ofNlrp3+/+orNlrp3−/−mice stained as infafter stereotaxic injection of vehicle or 25-HC. Scale bar, 100 μm. (h) Quantification of active caspase-3+oligodendrocytes in the confocal images of vehicle- or 25-HC-injected brain sections as treated ing. (n=6) (i) Quantification of active caspase-3+oligodendrocytes in the confocal images of vehicle- or 25-HC-injected brain sections ofAbcd1+/+(WT) orAbcd1−/−mice. (n=6) For all panels, *P<0.05, **P<0.01 and ***P<0.001. Figure 6: 25-HC promotes the microglial recruitment and oligodendrocyte cell death in an NLRP3 inflammasome-dependent manner. ( a ) Immunohistochemical staining of coronal brain sections with anti-Iba-1 antibody (green) and DAPI (blue) after bilateral stereotaxic injection of 25-HC (100 μM) or vehicle into the brain of Nlrp3 +/+ or Nlrp3 −/− mice. Scale bar, 200 μm. ( b ) Quantification of Iba-1 + microglia in confocal images of vehicle- or 25-HC-injected brains from Nlrp3 +/+ (WT) or Nlrp3 −/− (KO) mice. ( n =6). ( c ) Quantification of IL-1β in the brain homogenates of vehicle- or 25-HC-injected hemispheres from Nlrp3 +/+ (WT) or Nlrp3 −/− (KO) mice. ( n =7) ( d ) Immunohistochemical staining of brain sections with anti-Iba-1 antibody (green) after stereotaxic injection of 25-HC (100 μM) together with recombinant IL-1 receptor antagonist (IL-1Ra, 5 μg). Scale bar, 50 μm. ( e ) Quantification of Iba-1 + microglia in the confocal images of vehicle- or 25-HC-injected brain sections as treated in d . ( n =4) ( f ) Immunohistochemical staining of brain sections with anti-active caspase-3 antibody (green), anti-myelin basic protein antibody (MBP, red), and DAPI (blue). Lower panel is representative magnified image of a 25-HC-injected region. Arrows indicate the active caspase-3-positive oligodendrocytes (yellow). Scale bars, 200 μm (upper); 50 μm (lower). ( g ) Immunohistochemical staining of brain sections of Nlrp3 +/+ or Nlrp3 −/− mice stained as in f after stereotaxic injection of vehicle or 25-HC. Scale bar, 100 μm. ( h ) Quantification of active caspase-3 + oligodendrocytes in the confocal images of vehicle- or 25-HC-injected brain sections as treated in g . ( n =6) ( i ) Quantification of active caspase-3 + oligodendrocytes in the confocal images of vehicle- or 25-HC-injected brain sections of Abcd1 +/+ (WT) or Abcd1 −/− mice. ( n =6) For all panels, * P <0.05, ** P <0.01 and *** P <0.001. Full size image Oligodendrocytes are the major myelin-forming cells of the central nervous system. 25-HC injection caused robust apoptotic cell death of oligodendrocytes in the 25-HC-injected region, but not in the vehicle-injected contralateral region ( Fig. 6f ). This finding suggested that the increased level of 25-HC was indeed responsible for the depletion of oligodendrocytes; it is possible that oligodendrocyte depletion could lead to the demyelination observed in X-ALD. To our surprise, this 25-HC-induced loss of oligodendrocytes were significantly attenuated in Nlrp3 −/− mice ( Fig. 6g,h ). These findings clearly demonstrate that 25-HC could cause oligodendrocytes apoptosis via activation of the NLRP3 inflammasome. In support of our data, Abcd1 -deficient mice showed increased susceptibility to cerebral inflammations as shown by oligodendrocyte apoptosis ( Fig. 6i and Supplementary Fig. 18a ) and the recruitment of microglia ( Supplementary Fig. 18b,c ) in response to the stereotaxic administration of 25-HC. Our data collectively demonstrate that 25-HC promoted NLRP3 inflammasome assembly and activation that led to the recruitment of microglia and apoptosis of oligodendrocytes. The underlying mechanism by which cerebral inflammation is initiated has been a long-standing conundrum in the pathogenesis of X-ALD [7] . VLCFA is considered the best biomarker of X-ALD [6] , but its contribution to the neuroinflammation of CCALD is still unclear [10] . In the present study, we identified the unique upregulation of CH25H and the subsequent production of 25-HC in CCALD-derived cells. Indeed, accumulated VLCFA was responsible for the induction of CH25H ( Fig. 2f,g ). CH25H was previously suggested as a risk factor for the pathogenesis of Alzheimer’s diseases [37] , [38] , which indicated that CH25H induction and the subsequent production of 25-HC could contribute to the progression of neurodegenerative diseases. In correlation with this observation, our data showed that 25-HC could act as a potent mediator and inducer of cerebral inflammation in CCALD through its ability to activate the NLRP3 inflammasome. 25-HC was first identified as a feedback suppressor of cholesterol biosynthesis that acted mainly by inhibiting pathways involved with sterol response element-binding proteins [22] . CH25H is one of the highly inducible, interferon-stimulated genes expressed in response to viral infection [39] . Its product, 25-HC, affects multiple steps of the viral life cycle including the inhibition of viral entry, viral replication and particle assembly [23] , [39] . However, the contribution of 25-HC to the inflammatory response still remains to be further investigated, particularly in terms of transcriptional control of pro-inflammatory cytokine expressions. Previous literature reported that 25-HC could augment the inflammatory response, leading to increased secretion of pro-inflammatory cytokines, such as IL-1β and IL-6 (refs 40 , 41 , 42 , 43 ). Recently, Gold et al. showed that Ch25h −/− mice were less susceptible to influenza A virus infection due to a decreased inflammatory response, and proposed that 25-HC could amplify the production of toll-like receptor (TLR)-induced cytokines by facilitating AP-1-mediated transcription [40] . Supporting the pro-inflammatory role of 25-HC, another study demonstrated that 25-HC-triggered IL-1β production in co-cultures of human monocytes and vascular smooth muscle cells [41] . In correlation with its pro-inflammatory function, 25-HC has been considered to promote the progression of chronic inflammatory diseases, including atherosclerosis, chronic obstructive pulmonary disease, and Alzheimer’s disease [37] , [44] , [45] . However, the precise role of 25-HC in inflammasome activation at the molecular level has been poorly described to date. By contrast, a recent paper demonstrated increased secretion of IL-1β in Ch25h -deficient BMDMs upon LPS-ATP stimulation, and proposed that 25-HC could attenuate the production of pro-IL-1β by inhibiting sterol response element-binding proteins-mediated transcription [46] . We cannot fully explain these discrepancies about the contribution of 25-HC to inflammation at present. One possible explanation could be the different concentration of 25-HC used. For example, more than micromolar concentrations of 25-HC were employed in the studies proposing its pro-inflammatory action [40] , [41] , [42] , [43] , whereas nanomolar concentrations were used when documenting anti-inflammatory effects [46] . The physiological concentration of 25-HC in the brain is difficult to measure, but the level of 25-HC might possibly be elevated in the demyelinating plaque of CCALD due to the increased VLCFA level [47] , [48] . With these conflicting reports, we carefully examined the role of 25-HC in BMDMs, microglia, and human THP-1 cells, as well as in the mouse brain, and we provide definitive molecular evidences to support the pro-inflammatory role of 25-HC in NLRP3 inflammasome activation. Like other classical NLRP3 agonists, 25-HC also induced a potassium efflux-dependent NLRP3 inflammasome activation. Emerging evidence has proposed a potential linkage between mitochondrial damage or damaged mitochondria-derived danger signals such as mtROS and activation of the NLRP3 inflammasome under diverse stress conditions [33] , [49] . Of note, 25-HC caused robust production of mtROS and mitochondrial damage, which was consistent with the previous report [50] . The scavenging of mtROS markedly attenuated 25-HC-induced caspase-1 activation and ASC oligomerization under our experimental conditions. Despite the poor understanding of how 25-HC causes mitochondrial dysfunction, mitochondrial damage and mtROS were shown to be closely related to the pathogenesis of ALD [51] , [52] , [53] . In this regard, it is plausible that mtROS production is involved in 25-HC-induced NLRP3 inflammasome activation that could possibly result in the pathophysiology of CCALD. In addition, our data showed that 25-HC alone without LPS co-treatment could activate NLRP3 inflammasome in BMDMs and microglia, but failed to induce IL-1β mRNA expression. Considering that NLRP3 inflammasome activation requires a priming step, it is questionable as to whether 25-HC could provide a priming signal for NLRP3 activation in the physiological context. Of interest, 25-HC alone promoted NLRP3-independent cell death of BMDMs and mixed glial cells ( Supplementary Fig. 19 ), which suggested that 25-HC-triggered cell death could release a danger signal that functions as a priming signal under physiological conditions. Given that 25-HC is a potent ligand of the LXR pathways [25] , we also investigated the involvement of LXR signalling in 25-HC-triggered NLRP3 inflammasome activation. A recent report consistently demonstrated that LXR ligands could promote the activation of NLRP3 inflammasome in colon cancer cells leading to cell death [36] . In our study, LXR signalling was likely to be involved in the 25-HC-induced caspase-1 activation of BMDMs. However, whether the engagement of LXR is a potent stimulator of NLRP3 remains to be elucidated. Another LXR agonist, TO901317, showed potent caspase-1 activation in BMDMs, as well as in Nlrp3 -deficient cells. In this regard, further study will be required to address the precise role of the LXR pathways in inflammasome signalling. The potential contribution of the NLRP3 inflammasome to chronic inflammatory disorders has been increasingly demonstrated [54] . In correlation with our study, the NLRP3 inflammasome was already shown to play a crucial role in demyelination and oligodendrocyte loss in a mouse model [18] , which suggested the significance of the NLRP3 inflammasome in cerebral neuroinflammation. Interestingly, endogenous molecules such as palmitate, uric acid crystals, cholesterol crystals and amyloid β, which are critical in the pathogenesis of chronic metabolic or neurodegenerative disorders, have been shown to activate the NLRP3 inflammasome [13] , [54] . Here, we present evidence that 25-HC could act as an endogenous NLRP3 stimulator leading to cerebral inflammation. Therefore, our data suggest that therapeutic interventions that can target the NLRP3 inflammasomes may show clinical benefit for the treatment of X-ALD. Mice C57BL/6, Abcd1 +/− , and Nlrp3 −/− mice were obtained from The Jackson Laboratory and bred at Yonsei University College of medicine. All mice were on C57BL/6 background and 7–10 weeks male mice were used for the experiments. All mice were maintained under specific pathogen-free conditions. Protocols for the animal experiments were approved by the Institutional Ethical Committee, Yonsei University College of Medicine. All experiments were performed in accordance with the approved guidelines of the Institutional Ethical Committee. Establishment of X-ALD patients-derived cells hESC and human iPSCs were maintained as described previously [19] . Human X-ALD-fibroblasts (GM04496 (CCALD1), GM04934 (CCALD 3), GM04932 (CCALD4), GM07675 (AMN 2), GM17819 (AMN3)) and control human dermal fibroblast (HDF, C-004-5C) cells were purchased from Coriell Institute and Invitrogen, respectively. Human fibroblasts were cultured as recommended by the manufacturer. Human X-ALD-fibroblasts were also derived and established from skin punch biopsies taken from a Korean CCALD patient (CCALD 2) and Korean AMN patient (AMN 1). The patients’ clinical information is listed in the Supplementary Table 2 . Human iPSCs were established from control- (HDF), AMN3- and CCALD1-fibroblasts. Differentiation of oligodendrocytes was performed as described previously [19] and determined using anti-NG2 (Chemicon) and anti-A2B5 (Millipore) antibodies by flow cytometry. Ethical statement Yonsei University Institutional Review Board approval (IRB 4-2016-0194) was obtained for the generation and analyses of fibroblasts from adrenoleukodystrophy patients. All volunteers who participated in this study signed written informed consent forms before skin biopsy sampling for human fibroblast establishment. Cell cultures Mouse bone marrow cells were isolated from mouse femurs and differentiated into BMDMs with L929-conditioned medium [55] . Immortalized NLRP3-reconstituted BMDMs (N1-8) and NLRP3-GFP-expressing BMDMs were provided by E.S. Alnemri (Thomas Jefferson University, Philadelphia, PA, USA). All BMDMs were maintained in L929-conditioned DMEM supplemented with 10% FBS and antibiotics. THP-1 cells were differentiated into macrophage-like cells using a phorbol 12-myristate 13-acetate treatment and cultured in RPMI-1640 supplemented with 10% FBS, 2 mM glutamine, 10 mM HEPES, 1 mM sodium pyruvate, 0.05 mM 2-mercaptoethanol and antibiotics [56] . Mouse brain mixed glial cells were isolated from the whole brain of pups on the first postnatal day and cultured in DMEM/F-12 medium for 3 weeks as described previously [57] . Microglial cells were further enriched from the mixed glial cultures by mild trypsinization [58] . The microglia cultures were characterized by flow cytometry after co-staining with anti-CD11b and anti-F4/80 antibodies (eBioscience). Cell death was measured by the extracellular release of lactate dehydrogenase (LDH) using a CytoTox96 non-radioactive cytotoxicity assay kit (Promega). Microarray analysis Microarray analysis was performed by Macrogen Inc. Briefly, 200 ng of total RNA from purified hESCs (P35–45), control iPSCs (P10–20), CCALD-iPSCs (P10–20), AMN-iPSCs (P10–20) was transcribed to yield biotinylated complementary RNA according to the manufacturer’s instructions. Complementary RNA samples were each hybridized to a Human HT-12 v4.0 Expression Beadchip (Illumina). Arrays were scanned with an Illumina Bead Array Reader confocal scanner according to the manufacturer’s instructions. Raw data were processed using the Illumina GenomeStudio v2011.1 (Gene Expression Module v1.9.0)). Gene-enrichment and functional annotation analysis for the significant probe list was performed using Gene Ontology (www.geneontology.org/). All data analysis and visualization of differentially expressed genes was conducted using R 3.1.2 (www.r-project.org). Microarray data have been deposited in the Gene Expression Omnibus database (GSE85804). Measurement of VLCFA and 25-HC VLCFAs were measured as fatty acid methyl esters as described previously [19] . Briefly, after adding C27:0 as the internal standard, total lipid were extracted, converted to methyl esters, purified by thin-layer chromatography, and subjected to gas chromatography (GC). The level of 25-HC in culture media was determined by GC coupled with mass spectrometry (GC-MS) as described previously [59] . A deuterium-labelled internal standard (D6-25-HC) was used for calculating the concentration of 25-HC. ABCD1 expression To knockdown ABCD1 expression, cells were transfected with scrambled siRNA (4390843, Ambion) or ABCD1-targeting siRNAs (s1233, Invitrogen, 5′-CCUUCACUAUUGCCCGCAAtt-3′; 5′-UUGCGGGCAAUAGUGAAGGct-3′) using Lipofectamine RNAiMAX (Invitrogen) according to the manufacturer’s instructions. To induce ectopic expression of ABCD1 , cells were infected with lentiviral particles expressing vector or ABCD1. Lentiviral particles were prepared from the supernatants of 293GPG packaging cells transfected with empty or ABCD1 -expressing lentiviral construct (Addgene). Quantification of mRNA To measure mRNA production, total RNA was isolated using RNeasy Mini Kit (Intron) or Trizol reagent (Invitrogen) and reverse transcribed using Power cDNA synthesis kit (Intron). Quantitative real-time PCR were performed using SYBR Premix Ex Taq (Takara). Primers were as follows: (human CYP46A1 ) 5′-TGTGTTTTTGGATTG GGCTAAGA-3′ and 5′-ACTCAGGACTCGTGACGATGA-3′; (human CH25H ) 5′-GCACTGCCTGCCAAGCGAGA-3′ and 5′-CTCCGCAGACAGCTCCCCCT-3′; (human CYP27A1 ) 5′-CGGCAACGGAGCTTAGAGG-3′ and 5′-GGCATAGCCTTGAACGAACAG-3′; (mouse Cyp46a1 ) 5′-GGACATCTCCCCTACTTTTGGA-3′ and 5′-GGACCATACTTCTTAGCCCAATC-3′; (mouse Ch25h ) 5′-ATGGGCTGCTACAACGGTTC-3′ and 5′-CCTTGTCCTTATGGTGTCCCAG-3′; (mouse Cyp27a1 ) 5′-GCACAGGAGAGTACGGAGG-3′ and 5′-CGGGCAAGTGCAGCACATA-3′. Relative expression was expressed as means ± s.e.m. obtained from three independent experiments. Stereotaxic injection Mice were anaesthetized with a mixture of tiletamine/zolazepam (Zoletil) and xylazine (Rompun) and mounted in a stereotaxic frame (Stoelting). The mice were injected with vehicle or 25-HC in the white matter of the corpus callosum over both hemispheres (1 or −1 mm lateral to the midline, 1 mm anterior to Bregma and 2 mm deep) via separate Hamilton syringes. In some experiments, recombinant human IL-1Ra (5 μg, Prospec) was co-injected with 25-HC. After 3 days, mice were anaesthetized and were transcardially perfused with paraformaldehyde. Brains were removed and were placed overnight at 4 °C in 4% (vol/vol) paraformaldehyde, then transferred to PBS. Coronal sections of 20 μm in thickness were prepared using a Vibratome microtome (Leica). Immunohistochemistry Cells were fixed in 4% paraformaldehyde, permeabilized and stained with the primary antibodies targeting MBP (Abcam, ab7349, 1:100), cleaved caspase-3 (Cell Signaling Technology, 9661, 1:100) and Iba-1 (Wako, 019-19741, 1:100), followed by the appropriate Alexa Fluor 488- or 594-labelled secondary antibodies (Molecular Probes). DAPI counterstaining was used for nuclei visualization. Cell images were captured with an Olympus IX71 microscope and DP71 digital camera or Olympus FSX100 system. Iba-1-positive cells in the selected regions were counted using Image J. Immunoblot analysis Cells were lysed in buffer containing 20 mM HEPES (pH 7.5), 0.5% Nonidet P-40, 50 mM KCl, 150 mM NaCl, 1.5 mM MgCl 2 , 1 mM EGTA and protease inhibitors. Soluble lysates were fractionated by SDS–polyacrylamide gel electrophoresis and then transferred to polyvinylidene difluoride membranes. In some experiments, cell culture supernatants were precipitated by the addition of methanol/chloroform mixture as described previously [60] and then immunoblotted. The following antibodies were used for detecting mouse caspase-1 (Adipogen AG-20B-0042, 1:2,000), mouse IL-1β (R&D AF-401-NA, 1:1,000), human caspase-1 (Santa Cruz SC-515, 1:500), human IL-1β (Cell Signaling 2022, 1:1,000), mouse NLRP3 (Adipogen AG-20B-0014, 1:2,000) and mouse ASC (Santa Cruz SC-22514-R, 1:500). All the blots shown are representative image of at least three independent experiments. Images have been cropped for presentation. Full size images are presented in Supplementary Fig. 20 . Cytokine production assay The levels of IL-1β or IL-6 in the culture supernatants or the mouse brain homogenates were quantified by mouse IL-1β or IL-6 ELISA (R&D). For the brain homogenates, inflammatory cytokines were also quantified using the Cytometric Bead Array (CBA) Mouse Inflammatory Kit (BD). All the assay experiments were performed according to the manufacturer’s protocols. Assay of inflammasome/caspase-1 activation To induce a conventional NLRP3 inflammasome activation, BMDMs or microglial cells were primed with LPS (0.25 μg ml −1 , 3 h), followed with ATP treatment (2 ∼ 2.5 mM, 45 min). To measure the inflammasome-activating role of 25-HC or VLCFA, cells were treated with 25-HC (1 ∼ 100 μM) or VLCFA (up to 100 μM) for 10 h in the presence of LPS treatment (0.25 μg ml −1 , last 4 h). In some experiments, cells were first primed with LPS (0.25 μg ml −1 , 3 h), washed with PBS, and then treated with 25-HC or other agonists as indicated. Inflammasome activation was determined by the presence of active caspase-1 p20 (mouse BMDM) or p10 (human THP-1 cells), and active IL-1β from culture supernatants in immunoblots, and by the extracellular IL-1β quantification using ELISA. FAM-FLICA-caspase-1 assay kit (ImmunoChemistry) was employed to detect active caspase-1 in the brain sections according to the manufacturer’s protocol. Assay of NLRP3 inflammasome assembly To measure the oligomerization of NLRP3, confocal microscopy of NLRP3-GFP-expressing BMDMs was performed as described previously [61] . To quantify NLRP3 speck formation, the relative percentage of NLRP speck-containing cells was determined by dividing the number of NLRP3 speck-containing cells by the number of total cells. To determine the oligomerization of ASC, DSS-mediated crosslinking assay was performed as described previously [62] . To visualize the molecular interaction of NLRP3 with ASC, proximity-ligation assay was performed using Duolink In Situ Red starter kit (Sigma) using anti-ASC or anti-NLRP3 antibodies according to the manufacturer’s protocols. The relative proximity-ligation signals (PL signals/DAPI signals) were quantified using Image J and calculated as a relative fold-change compared with untreated controls. Measurement of mitochondrial ROS and damage To measure mROS production, cells were stained with MitoSOX (Invitrogen) according to the manufacturer’s protocol and the fluorescence of the cells was then monitored and analysed by flow cytometry (FACSVerse, BD). To assess mitochondrial membrane potential-dependent damage, cells were co-stained with MitoTracker Deep Red and MitoTracker Green (Invitrogen) according to the manufacturer’s protocol and analysed by flow cytometry. All flow cytometry data are representative of at least three independent experiments. Statistical analysis All values are expressed as the mean±s.e.m. of individual samples or independent experiments. Data were analysed using the Student’s t test, and P values≤0.05 were considered significant. Data availability Microarray data that support the findings of this study have been deposited in the Gene Expression Omnibus (GEO) database with the accession code GSE85804 . How to cite this article: Jang, J. et al. 25-hydroxycholesterol contributes to cerebral inflammation of X-linked adrenoleukodystrophy through activation of the NLRP3 inflammasome. Nat. Commun. 7 , 13129 doi: 10.1038/ncomms13129 (2016).